Optical switching of nuclear spin–spin couplings in semiconductors Two-qubit operation is an essential part of quantum computation. However, solid-state nuclear magnetic resonance quantum computing has not been able to fully implement this functionality, because it requires a switchable inter-qubit coupling that controls the time evolutions of entanglements. Nuclear dipolar coupling is beneficial in that it is present whenever nuclear–spin qubits are close to each other, while it complicates two-qubit operation because the qubits must remain decoupled to prevent unwanted couplings. Here we introduce optically controllable internuclear coupling in semiconductors. The coupling strength can be adjusted externally through light power and even allows on/off switching. This feature provides a simple way of switching inter-qubit couplings in semiconductor-based quantum computers. In addition, its long reach compared with nuclear dipolar couplings allows a variety of options for arranging qubits, as they need not be next to each other to secure couplings. Nuclear magnetic resonance (NMR) quantum computing has attracted broad interest because it is one of the most advanced testbeds for quantum computation. Although the interest began with solution NMR [1] , [2] , [3] , it is now believed that scalable NMR quantum computers in the future will be built on semiconductors based on highly developed semiconductor technology [4] , [5] , [6] . The main challenges include the initialization and the creation of spin entanglement, which are essential features of quantum computation [7] . Semiconductor-based NMR quantum computers are advantageous as they can be achieved optically; that is, the initialization (nuclear–spin polarization) is provided by optical pumping [8] , [9] , and the entanglement is created via internuclear (nuclear spin–spin) couplings between polarized nuclei [10] , [11] . In optically pumped semiconductors, the latter manifests itself as dipolar order [12] , [13] and double-quantum coherence [14] . Switchability is another essential functionality required for internuclear couplings, which should be 'on' during operations and 'off' otherwise. In this respect, nuclear dipolar coupling ( D- coupling, hereafter) is not the best choice for the above-mentioned reasons. In addition, the time required for operations increases rapidly with increasing qubit number because of decoupling operations [15] . Other possible candidates include indirect couplings mediated by donor electrons [4] and magnons [15] . Their implementations are fairly challenging, however, given the complicated switching mechanisms. By contrast, the scheme presented in this paper is rather simple; the coupling strength can be controlled externally through light power, and on/off switching can be easily implemented. In this study, we have preformed cross-polarization (CP) experiments with GaAs under light illumination, and demonstrated that a nuclear spin–spin coupling grows in strength, and extends its reach to farther nuclei as light power is increased. These futures bring about a unique transition of the CP process from oscillatory behaviour in the 'dark' towards exponential relaxation with increasing light power. The experiments provide us with information on the essential features of the optically induced nuclear spin–spin couplings; in particular, we find that the coupling strength is roughly proportional to light power, which is essential for the switching of the couplings. CP process in GaAs in the dark The present mechanism is manifested in a CP process from 75 As ( I -spin) to 71 Ga ( S -spin) in GaAs under infrared light irradiation. Before detailing this process, we first describe it in the dark (without light irradiation) as a reference. This is an ordinary CP process, for which we expect a contact time ( cp ) dependence of S -magnetization ( M S eq ) of the form where T IS is the cross-relaxation time. A relaxation process in the rotation frame ( T 1ρ ) need not be considered here, as it is sufficiently long because of high crystal symmetry [16] , [17] . The reality, however, is more complicated than equation (1). 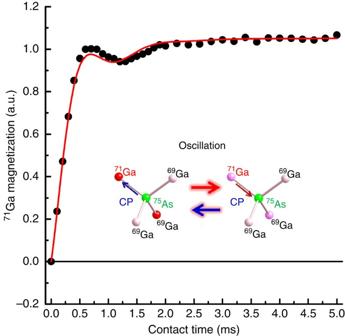Figure 1: CP experiment in GaAs in the dark. Contact time (cp) dependence of71Ga magnetization (MSeq) in a cross polarization experiment in the dark at 10 K, normalized atcp=0.7 ms. The pulse sequence is shown inFigure 5, where the light is turned off, that is,PIR=0 mW. The magnetization is transferred back and forth between75As and71Ga at a nearest neighbour site. This process gives rise to a transient oscillation. The solid red line represents the best-fit curve using equation (2). Figure 1 shows M S eq ( cp ) obtained in the dark, which exhibits a clear transient oscillation. Figure 1: CP experiment in GaAs in the dark. Contact time ( cp ) dependence of 71 Ga magnetization ( M S eq ) in a cross polarization experiment in the dark at 10 K, normalized at cp =0.7 ms. The pulse sequence is shown in Figure 5 , where the light is turned off, that is, P IR =0 mW. The magnetization is transferred back and forth between 75 As and 71 Ga at a nearest neighbour site. This process gives rise to a transient oscillation. 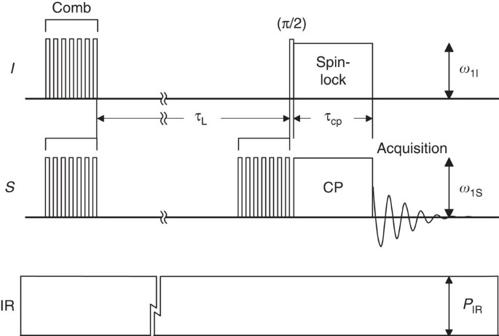Figure 5: Pulse sequence. Pulse sequence for optical pumping CP experiments.I=75As,S=71Ga and IR=infrared light (1.50 eV, σ−). 'Comb': comb pulse consisting of a number of π/2 pulses.L: duration of light irradiation (=60 s).cp: contact time for CP.ω1I/2π,ω1S/2π: rf-pulse strengths in terms of Rabi frequency (=35 kHz).PIR: infrared light power. The horizontal axis is not to scale. The solid red line represents the best-fit curve using equation (2). Full size image Transient oscillations have been reported in some molecular crystals, and attributed to discrete S–I coupling spectra of isolated S–I pairs [18] , [19] , [20] . The magnetization is transferred back and forth inside the pair with a frequency corresponding to half the flip-flop term of the D -coupling. The present sample, however, is not a molecular crystal, so isolated pairs are expected to be rare. Here an essential factor is the existence of two Ga isotopes, that is, 69 Ga and 71 Ga with natural abundances of 69 N A =0.604 and 71 N A =0.396, respectively. A local 75 As - 71 Ga pair appears when only one of the four nearest-neighbour sites of 75 As is occupied by 71 Ga and the others are occupied by 69 Ga. The probability of finding such pairs is 4 C 1 · 71 N A ·( 69 N A ) 3 =0.35; that is, about 35% of 75 As have a single 71 Ga in the vicinity and contribute to the oscillation. The pairs are coupled through indirect scalar coupling J IS , where D -couplings are absent because the Ga sites are situated at magic angle positions in the (100) crystal orientation [16] , [17] , [21] . The process is described by a damping oscillation [18] , where Ω is the oscillation frequency (Ω= J IS /2) and R is the damping factor. We fit the data using equation (2) with Ω and R as free parameters. The best result is obtained with Ω=0.74 kHz, which yields J IS =2Ω=1.48 kHz. This value is comparable with that in the InP case ( J IS =2.3 kHz) [17] . The fitting curve is shown by a solid line in Figure 1 . 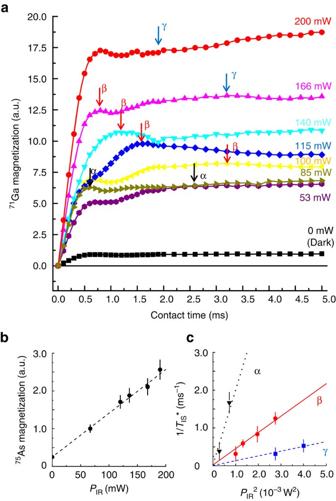The fit is not very good at the beginning of the oscillation; this may be due to the presence of 75 As sites with more than one 71 Ga nucleus in the four nearest-neighbour sites. Figure 2: CP experiments in GaAs under light irradiation. (a) Contact time (cp) dependence of71Ga magnetization (Ms) in CP experiments at 10 K measured under light irradiation with powerPIRranging from 0 to 200 mW. The pulse sequence is shown inFigure 5. The data atPIR=0 mW are the same as those inFigure 1. Black, red and blue arrows represent the three series of maxima. (b) The light power (PIR) dependence of75As magnetization (MI), which represents the enhancement of the nuclear spin polarization due to the optical pumping effect. The magnetization exhibits a linear dependence withPIR. The error bars represent the data scatterings in a few experiments performed under the same conditions. (c) The values offor the three series (α, β and γ) marked by the arrows in (a) plotted against. The error bars represent the breadth around each peak. The lines are visual guides. CP process under light irradiation Figure 2a shows the cp dependence of S -polarization, M S ( cp ) under various levels of light power, P IR , which exhibits new local maxima (peaks) that are not observed in the dark. The maxima form a number of series (α, β, γ...), and the maximal position in each series shifts towards smaller values of cp as the light power is increased. For example, the series 'β' shown by the red arrows starts with a broad maximum around cp =3.1 ms at P IR =100 mW, which shifts towards smaller values of cp as P IR is increased and eventually merges into a peak at cp =0.8 ms at 166 mW. 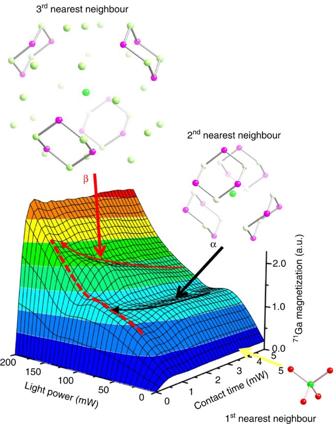These maxima represent new polarization transfer processes that appear under light irradiation. Figure 3: Light power dependence of the CP process in GaAs. Three-dimensional representation ofFigure 2aobtained by interpolating the data in between. The data shown by the yellow arrow represents those in the dark (PIR=0 mW), which corresponds to the polarization transfer to the nearest-neighbour71Ga through the conventionalJIS. The black (α) and red (β) arrows indicate the series of maxima corresponding, presumably, to the polarization transfers to the second and third nearest neighbour sites, respectively. The dotted red line represents the71Ga magnetization atcp=0.7 ms, which exhibits a plateau-like feature (that is, less steeper slope) around 80 mW. Figure 3 shows a three-dimensional representation of Figure 2a obtained by interpolating the data in between. The continuous shift of the maximum in each series can be readily confirmed. Figure 2: CP experiments in GaAs under light irradiation. ( a ) Contact time ( cp ) dependence of 71 Ga magnetization ( M s ) in CP experiments at 10 K measured under light irradiation with power P IR ranging from 0 to 200 mW. The pulse sequence is shown in Figure 5 . The data at P IR =0 mW are the same as those in Figure 1 . Black, red and blue arrows represent the three series of maxima. ( b ) The light power ( P IR ) dependence of 75 As magnetization ( M I ), which represents the enhancement of the nuclear spin polarization due to the optical pumping effect. The magnetization exhibits a linear dependence with P IR . The error bars represent the data scatterings in a few experiments performed under the same conditions. ( c ) The values of for the three series (α, β and γ) marked by the arrows in ( a ) plotted against . The error bars represent the breadth around each peak. The lines are visual guides. Full size image Figure 3: Light power dependence of the CP process in GaAs. Three-dimensional representation of Figure 2a obtained by interpolating the data in between. The data shown by the yellow arrow represents those in the dark ( P IR =0 mW), which corresponds to the polarization transfer to the nearest-neighbour 71 Ga through the conventional J IS . The black (α) and red (β) arrows indicate the series of maxima corresponding, presumably, to the polarization transfers to the second and third nearest neighbour sites, respectively. The dotted red line represents the 71 Ga magnetization at cp =0.7 ms, which exhibits a plateau-like feature (that is, less steeper slope) around 80 mW. Full size image This phenomenon can be explained by discrete increments in the number of S -nuclei ( 71 Ga) involved: in the dark ( P IR =0 mW), the number of nuclei participating in the process is small and oscillatory behaviour is observed, as shown in Figure 1 . Light illumination causes a series of S -nuclei batches (α, β, γ...) to participate in sequence. Their contributions are successively added to the signal intensity one after another, whereas the speed of transfer from I - to S -nuclei in each series increases with the light power (that is, the maximal position shifts towards smaller values of cp ). As the number of nuclei involved is further increased, the cross relaxation is expected to approach the exponential relaxation behaviour given by equation (1) [20] . That is, we see here the transition from oscillatory behaviour in the 'dark' towards exponential relaxation with increasing light power. This is a unique case in that such a transition can hardly be observed in ordinary NMR measurements. Another factor responsible for the phenomenon is the optical pumping effect [8] , [9] . It contributes to the S -magnetization ( 71 Ga) through the enhancement of the I -magnetization ( 75 As) caused by the polarization transfer from the optically oriented electrons for the duration of light irradiation L =60 s. Figure 2b shows the light-power dependence of the I -magnetization ( 75 As), which increases linearly with light power. This enhancement is partly responsible for the increase of the S -magnetization with increasing light power, as seen in Figures 2a and 3 . The cp dependence of M s is expressed as, where M I dark ( L ) in the first term on the right-hand side represents the I -magnetization in the dark portion of the sample recovered during L =60 s and represents the polarization transfer process to S- spins in the first nearest neighbour sites through J IS . This process is essentially the same as that in Figure 1 . On the other hand, in the second term is the I -magnetization in the illuminated area generated by the optical pumping effect during L =60 s, whose P IR dependence is shown in Figure 2b . This magnetization is transferred to S -spins through the two processes shown in the brackets: the same process as that in the dark, , and additional ones induced by light irradiation, . The latter are caused by the optically induced heteronuclear indirect coupling, . We will discuss characteristics of this coupling in the next section. The new coupling is presumably mediated by photo-excited electrons. It is known that electrons in metals can mediate indirect nuclear spin–spin couplings, a process referred to as the RKKY interaction [22] . In the present case, however, is observed in semiconductors where no intrinsic Fermi surfaces exist. Moreover, the lifetimes and spin relaxation times of the photo-excited electrons usually fall in the range between pico- and nanoseconds, which is more than six orders of magnitude smaller than that of the CP process, that is, milliseconds. It is intriguing that two phenomena with such different time scales are coupled with each other. The strength of in each batch (α, β, γ...) can be evaluated by the cross-relaxation time T IS opt in . According to Demco et al . [17] , [20] , [23] , the cross-relaxation time is expressed as where c is the correlation time of the CP and, is the second moment of the I–S heteronuclear spectrum due to . Equation (5) indicates that M 2 IS is proportional to ( ) 2 . Provided that is proportional to P IR and that c is independent of , equations (4) and (5) lead to the conclusion that 1/ T IS opt is proportional to P IR 2 . The actual value of T IS opt in each batch is determined from the analysis of the functional form of . Here we evaluate it from the maximal position; T IS * is defined as the contact time at which the maximum is formed. Figure 2c shows 1/ T IS * for the three series of maxima (α, β and γ) plotted against P IR 2 . The graph suggests that 1/ T IS * is roughly proportional to P IR 2 , implying that is proportional to P IR . This result provides a clue to the nature of the series of S -nuclei batches (α, β, γ...). Equation (5) indicates that the condition is fulfilled only when all I–S pairs participating in the summation of the right-hand side share the same , such that can be taken out of the summation Σ. Therefore, each series may be assigned to the polarization transfers to a batch of S -spins at the same distance from the I -spin at the origin. Figure 3 illustrates this situation. For example, the α-maxima may be assigned to the second nearest-neighbour S -spins, the β-maxima to the third, and so forth. It is reasonable that equivalent S -spins in the same order situated at the same distance from the I -spin share the same scalar coupling with it. Moreover, the contributions from nuclei in the same order to the correlation time are partially cancelled out [17] , [20] , [23] . Therefore, the assumption that c is independent of may be a reasonable approximation. The result also provides us with information about the reach of . The dotted red line in Figure 3 shows the P IR dependence of M s ( cp ) at a constant cp . One finds a plateau-like feature around 80 mW, which indicates that the S- spins at the third nearest-neighbour sites participate in the process only when P IR >80 mW; that is, can reach farther than D- and J IS -couplings, as the latter two may not substantially reach the third-nearest neighbours. 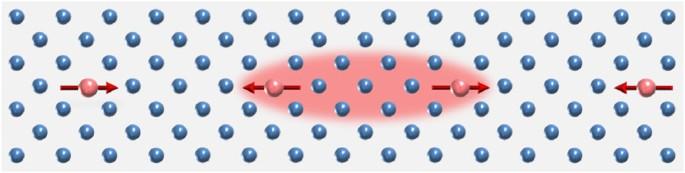Features such as the external switchability and the long reach may add variety to the qubit arrangement in semiconductor-based NMR quantum computers. Figure 4: Optical switching of a nuclear spin–spin coupling. A conceptual (ideal) model of optical switching of a nuclear spin–spin coupling between nuclear–spin qubits (red arrows) spaced a few lattice points apart from each other. Blue balls represent 'inert' (for example, spin-zero) nuclei. The nuclear dipolar couplings between the qubits are out of reach. Once the light is illuminated, a coupling emerges between the qubits. The strength of the coupling can be controlled externally through light power. Figure 4 shows an example. In an array of nuclear–spin qubits, a few lattice points apart from each other, the D -couplings are out of reach, so that the qubits are decoupled. Then, the present mechanism provides the external control of internuclear couplings. As the light power is increased, the reach of couplings is extended. This would further enhance the flexibility of qubit arrangements. Figure 4: Optical switching of a nuclear spin–spin coupling. A conceptual (ideal) model of optical switching of a nuclear spin–spin coupling between nuclear–spin qubits (red arrows) spaced a few lattice points apart from each other. Blue balls represent 'inert' (for example, spin-zero) nuclei. The nuclear dipolar couplings between the qubits are out of reach. Once the light is illuminated, a coupling emerges between the qubits. The strength of the coupling can be controlled externally through light power. Full size image This mechanism is compatible with most schemes proposed for semiconductor-based NMR quantum computing. The implantation of nuclear spin arrays in semiconductors has been studied using various techniques such as scanning probe microscopes, ion beams, and isotope engineerings [24] , [25] , [26] . These techniques will provide promising technologies to implement the schemes shown in Figure 4 . In conclusion, we have discovered an optically switchable indirect nuclear spin–spin coupling, which is manifested in CP experiments with GaAs under light illumination. As the strength of this coupling is externally controllable through light power, we expect it to have an essential role in the quantum gate operations of solid-state NMR quantum computers in the future. Optical pumping double resonance NMR system and the sample The CP experiments were performed at 10 K using an optical-pumping double-resonance NMR system developed for this study. The system consists of an NMR spectrometer, a laser system and a cryostat loaded in a 6.34-T superconducting magnet. A custom-built double-resonance probe is installed inside the cryostat. The sample used in this study is an undoped semi-insulating GaAs single-crystal wafer with a thickness of 600 μm and a crystal orientation of (100) (Mitsubishi Chemical). It is mounted on a sample stage made of sapphire located at the probe head and set with the surface normal to the magnetic field. The sample stage is cooled through thermal contact with the cold head of the cryostat. Infrared light emitted from a Ti:Sapphire laser is delivered to the cryostat through a polarization-maintaining fibre [27] . It is converted to circularly polarized light by a quarter-wave plate at the probe head, and applied to the sample in parallel to the magnetic field. The spot size at the sample surface is about φ 5 mm. Pulse sequence The pulse sequence used is shown in Figure 5 . The magnetization of I -spins, saturated by the first comb pulse, is regenerated during the time interval L and transferred to S- spins through the CP immediately thereafter. The infrared light is irradiated at a constant strength P IR throughout the sequence. The photon energy of 1.50 eV (near the band gap) and the helicity σ − were selected so that the optical pumping NMR signal enhancements for both 71 Ga and 75 As were nearly maximal. The experiment in the dark ( Fig. 1 ) was obtained with the same pulse sequence as that in Figure 5 , with the exception that P IR =0 mW. Figure 5: Pulse sequence. Pulse sequence for optical pumping CP experiments. I = 75 As, S = 71 Ga and IR=infrared light (1.50 eV, σ − ). 'Comb': comb pulse consisting of a number of π/2 pulses. L : duration of light irradiation (=60 s). cp : contact time for CP. ω 1I /2π, ω 1S /2π: rf-pulse strengths in terms of Rabi frequency (=35 kHz). P IR : infrared light power. The horizontal axis is not to scale. Full size image How to cite this article: Goto, A. et al . Optical switching of nuclear spin–spin couplings in semiconductors. Nat. Commun. 2:378 doi: 10.1038/ncomms1378 (2011).